Peptidoglycan architecture can specify division planes inStaphylococcus aureus Staphylococci are known to divide sequentially on orthogonal planes in three dimensions [1] : in a 3D Cartesian coordinate system with axes x , y and z , cells might divide in the x – y plane, then the x – z plane, then the y – z plane. This division schema, coupled with incomplete cell separation, results in the 'bunch of grapes' structure of clusters of cells for which the genus was originally named [2] . The resulting juxtaposition of cells presumably enhances the ability of Staphylococci to exploit their evolutionary niche. The organisms are further constrained to divide equatorially, with each daughter cell inheriting half of the parent, and to ensure that daughter nucleoids are correctly positioned and not damaged by the closing septum. Equatorial division is a characteristic common to vegetative bacterial cells in many genera; protection of nucleoids is universally required for correct inheritance of genetic information, and the core mechanisms by which these are achieved may well be conserved across a wide range of species. Division in more than one plane is less common and has been observed to take at least three forms: division in three orthogonal planes (for example, Staphylococcus , Sarcina [3] ), division in two specific orthogonal planes (for example, Pediococcus [3] ) or division in sequentially orthogonal planes, but with a degree of rotational freedom (for example, Escherichia coli Δ rodA mutant [4] , [5] ). S. aureus must 'remember' the planes of the previous two divisions in order to divide with fidelity, these spatial data are modified with each division and so cannot be encoded by DNA. We are compelled to assume the existence of heterogeneity in the spatial distribution of non-DNA cell components that either template septum formation or mark the location of previous division planes. The importance of such epigenetic information in cell cortex [6] , membrane [7] , [8] and prion [9] structure is well established. One cellular structure has not previously been considered to have a potential role in defining the division plane. Cellular morphology in most bacteria is maintained by an envelope of peptidoglycan, the chemical structure of which is well known [10] , [11] . Peptidoglycan is conserved over a wide range of cell shapes (for example, spheres, spirals, rods). In the absence of a cell wall, turgor pressure drives the cell towards the most energetically favourable conformation; a sphere [12] . Two possible paradigms for the nanoscale arrangement of glycan strands, the peptidoglycan structure, have been proposed: arrangement of glycan strands in the plane of the cytoplasmic membrane [13] or in a scaffold perpendicular to the cytoplasmic membrane [14] , [15] . The glycan chain lengths in S. aureus are sufficiently short to permit either of these configurations [16] . However, the planar orientation is adopted in the rod-shaped Gram-negative organisms E. coli and Caulobacter crescentus [17] and the rod shaped Gram-positive Bacillus subtilis has a more complex architecture with apparent helices of very long glycan strands [18] . Most microscopic observations with nanoscale resolution of the cell wall in S. aureus have been obtained on whole or living cells in which the peptidoglycan structure may be obscured by proteins and teichoic acids. These observations show that S. aureus are generally spherical, but adjacent pseudo-hemispherical cells have been observed [3] , [19] as the result of a recent division. Smooth and concentric ring-banded surface textures have been observed by electron microscopy of whole cells [3] and purified sacculi [20] . The ring-banded surface is attributed to septal peptidoglycan and may be indicative of the alignment of glycan strands in the bulk material or of scarring resulting from the action of autolysins that split daughter cells [3] . These surface structures have been seen in atomic force microscopy (AFM) images of living S. aureus [21] , as has an additional 'network' or 'honeycomb' surface arrangement [21] , [22] , [23] . Sections viewed by transmission electron microscopy show that spherical cells are completely bisected by the septal disc before splitting [3] , [21] . Equatorial rings have been observed by scanning electron microscopy of purified sacculi [24] . Here, we have used AFM imaging of purified S. aureus peptidoglycan sacculi to identify surface architectural features revealing the arrangement of peptidoglycan, including nanoscale surface textural features and larger bands of material, which would span the cells. The distribution of nascent peptidoglycan has been correlated with cell shape, size and relative juxtaposition using fluorescent vancomycin labelling and optical microscopy. These data are used to inform a consensus model of the architecture of S. aureus peptidoglycan throughout the cell cycle. We have identified features in peptidoglycan that demark previous divisions and, in doing so, hold the necessary information to specify the next division plane. We propose that the information is used by the organism for this purpose, by a currently unknown mechanism. Large-scale morphology of peptidoglycan To conduct sacculus analysis of S. aureus , cells were broken by gentle physical shearing and purified using SDS to remove cytoplasmic material and lipids, pronase to remove covalently linked cell wall proteins and hydrofluoric acid to remove teichoic acids [11] . This method of purification is generally accepted to leave the unstressed peptidoglycan chemically unaffected and constitutes the minimum possible treatment required to ensure that the subject of our microscopic investigations is peptidoglycan. In excess of 400 images of sacculi were obtained by tapping-mode AFM, set to acquire both height and phase signals. The height signal shows the topography of the sample, whereas the phase signal, although often highlighting topographic features, conflates these with variations in the adhesive and mechanical properties of the sample. The features we refer to here are present in both height and phase, but are often harder to distinguish in height. The random deposition of material on the mica substrate allowed intact and broken sacculi to be observed in a range of orientations ( Fig. 1a ). However, in cases in which cells were not broken and retained their cytoplasmic contents, surface features were obscured ( Fig. 1a and Supplementary Fig. S1 ). 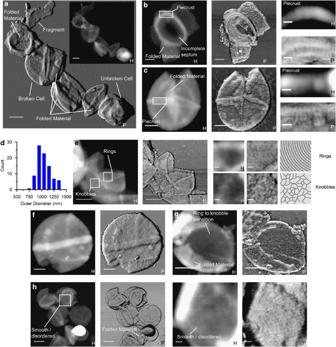Figure 1:S. aureuspeptidoglycan sacculus architecture. AFM height (H) and phase (P) images of purified sacculi from exponential phaseS. aureuswith interpretive diagrams, where appropriate. (a) Field showing sacculi of broken and unbroken cells. (b) Sacculus showing apparent incomplete septum, parallel to the plane of the image, encircled by a piecrust feature associated with the initiation of septum formation; inset shows detail of piecrust features. (c) Sacculus with a piecrust feature folded onto the plane of the image; inset shows details of piecrust feature. (d) Histogram showing measurements of the outer diameter of the piecrust (n=89 sacculi) as measured from AFM images in which the piecrust is in the plane of the mica substrate, showing that it does not contract to form an annulus and is therefore associated not with the leading edge of the septum but with the lagging edge. (e) Sacculus showing ring texture associated with nascent peptidoglycan and knobble texture associated with older peptidoglycan; insets show details of rings and knobbles. (f) Sacculus showing an intact disc of material with a faint ring structure surrounded by knobble structures. (g) Sacculus fragment showing presumed transition from ring to knobble surface texture. (h) Sacculus from a stationary phase culture showing smoother structure, less ordered than exponential phase without overt rings or knobbles; inset (right) shows details from marked region ofh. Scales: (a) bar 500 nm, H 200 nm, P 16°; (b) bar 250 nm, H 100 nm, P 9°, inset bar 50 nm, H 12.5 nm, P 9°; (c) bar 250 nm, H 75 nm, P 13°, inset bar 50 nm, H 12.5 nm, P 13°; (d) histogram; (e) bar 500 nm, H 100 nm, P 9°, inset rings bar 50 nm, H 18 nm, P 9°, inset knobbles bar 50 nm, H 20 nm, P 9°; (f) bar 250 nm, H 75 nm, P 6°; (g) bar 500 nm, H 50 nm, P 35°; (h) bar 500 nm, H 150 nm, P 12°, inset bar 50 nm, H 20 nm, P 6°. Figure 1: S. aureus peptidoglycan sacculus architecture. AFM height (H) and phase (P) images of purified sacculi from exponential phase S. aureus with interpretive diagrams, where appropriate. ( a ) Field showing sacculi of broken and unbroken cells. ( b ) Sacculus showing apparent incomplete septum, parallel to the plane of the image, encircled by a piecrust feature associated with the initiation of septum formation; inset shows detail of piecrust features. ( c ) Sacculus with a piecrust feature folded onto the plane of the image; inset shows details of piecrust feature. ( d ) Histogram showing measurements of the outer diameter of the piecrust ( n =89 sacculi) as measured from AFM images in which the piecrust is in the plane of the mica substrate, showing that it does not contract to form an annulus and is therefore associated not with the leading edge of the septum but with the lagging edge. ( e ) Sacculus showing ring texture associated with nascent peptidoglycan and knobble texture associated with older peptidoglycan; insets show details of rings and knobbles. ( f ) Sacculus showing an intact disc of material with a faint ring structure surrounded by knobble structures. ( g ) Sacculus fragment showing presumed transition from ring to knobble surface texture. ( h ) Sacculus from a stationary phase culture showing smoother structure, less ordered than exponential phase without overt rings or knobbles; inset (right) shows details from marked region of h . Scales: ( a ) bar 500 nm, H 200 nm, P 16°; ( b ) bar 250 nm, H 100 nm, P 9°, inset bar 50 nm, H 12.5 nm, P 9°; ( c ) bar 250 nm, H 75 nm, P 13°, inset bar 50 nm, H 12.5 nm, P 13°; ( d ) histogram; ( e ) bar 500 nm, H 100 nm, P 9°, inset rings bar 50 nm, H 18 nm, P 9°, inset knobbles bar 50 nm, H 20 nm, P 9°; ( f ) bar 250 nm, H 75 nm, P 6°; ( g ) bar 500 nm, H 50 nm, P 35°; ( h ) bar 500 nm, H 150 nm, P 12°, inset bar 50 nm, H 20 nm, P 6°. Full size image Thick bands of material, often exhibiting a corrugated 'piecrust' texture, were observed either as circles in the plane of the mica ( Fig. 1b ) or folded into lines at orientations, indicating that they would encircle intact cells ( Fig. 1c ). These are obviously distinct from folds in the sacculi that take the form of circular arcs (annotated throughout Fig. 1 ) and have previously been observed in other species [25] . Two orthogonal bands were often visible, one less distinct than the other ( Fig. 1 and Supplementary Fig. S1 ). The less-distinct bands, ribs, are thought to be the remnants of thick piecrusts from previous divisions. Similar structures were observed by transmission electron microscopy ( Supplementary Fig. S2 ). Incomplete septa were occasionally observed and each was surrounded by a thick piecrust band of material ( Fig. 1b and Supplementary Fig. S3 ). This is a strong indication that the piecrust forms before centripetal assembly of the septal disc. The outer diameter of piecrust bands of material enclosing continuous cell wall was measured to be 1,100 nm (s.d. 100 nm, n =89, Fig. 1d ), slightly smaller than the diameter of fixed cells measured from optical micrographs of 1,400 nm (s.d. 200 nm, n =127). Nanoscale architecture Of 328 identified sacculi or fragments from exponential phase cultures, 4% exhibited concentric ring-banded surface textures and 56% exhibited knobbly surface textures ( Fig. 1e,f and Supplementary Fig. S4 ). Concentric ring structures are associated with nascent peptidoglycan, as they have previously been visualized on opposing adjacent surfaces of newly divided sister cells by electron microscopy [3] , [26] . Here, similar structures were identified covering less than half of the sacculi and enclosed by a thicker band of material. Rarely observed were regions of peptidoglycan expressing a hybrid of the ring and knobble architecture ( Fig. 1g and Supplementary Fig. S4 ). Smoother surfaces, less ordered than those in cells from exponential phase, were generally observed in purified sacculi of stationary phase cells ( Fig. 1h ), likely due to gradual erosion of the ordered material by further autolysis. Remodelling of peptidoglycan during the cell cycle To correlate the morphologies observed by AFM with the cell cycle-associated peptidoglycan dynamics, S. aureus were monitored by vancomycin-BODIPY FL labelling of nascent peptidoglycan [27] . Fluorescence and differential interference contrast images were analysed and cells were characterized to yield novel information on cell cycle dynamics. S. aureus were grown in brain heart infusion (BHI) broth containing 125 mM D-serine, BHI (Ser+), with a transient incubation in BHI broth without D-serine, BHI (Ser−). We also discovered that pulse labelling of peptidoglycan can be achieved by this means. Nascent peptidoglycan was observed as a ring or disc in a plane bisecting the organism, the septum ( Fig. 2 ), corollary with a previous study [27] . Our AFM data indicate that the structure of this material would initially be concentric rings. Further to this, pairs of sister cells were observed that had partially separated with nascent peptidoglycan forming pseudo-hemispheres ( Fig. 2 ). Some such cells exhibited staining in a partially split (Y) conformation, indicating that autolysis of the surface had not occurred all along the outside of the septal disc. 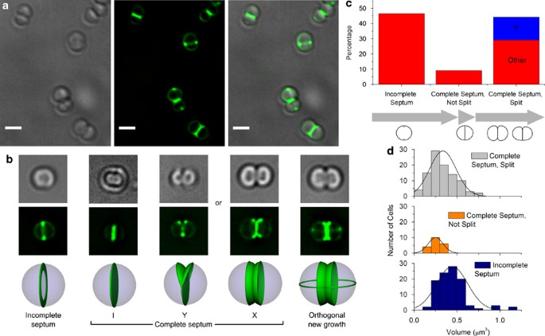Figure 2: Cell cycle-associated peptidoglycan and morphological dynamics inS. aureus. S. aureuswere grown in BHI (Ser +); nascent peptidoglycan was labelled with fluorescent vancomycin after 25 min of growth in BHI (Ser−). (a) Field showing several cells (left panel differential interference contrast, middle panel fluorescence, right panel combined, scale bar 1 μm). (b) Archetypical cell shapes and septum location during division; I=staining of septal disc, Y=staining of septum split into a Y shape, X=staining of septum split into an X shape. Top row: differential interference contrast images, middle row: fluorescence images, lower row: interpretive diagrams. Images have been rotated for ease of comparison. (c) Percentages of organisms exhibiting incomplete or complete septa, or complete split septa (n=219, organisms either isolated or coadhered in pairs; other: staining in an X or indistinct shape). (d) Cell volume in relation to splitting and septal state—newly septated cells that are yet to split have a lower volume than others. Figure 2: Cell cycle-associated peptidoglycan and morphological dynamics in S. aureus . S. aureus were grown in BHI (Ser +); nascent peptidoglycan was labelled with fluorescent vancomycin after 25 min of growth in BHI (Ser−). ( a ) Field showing several cells (left panel differential interference contrast, middle panel fluorescence, right panel combined, scale bar 1 μm). ( b ) Archetypical cell shapes and septum location during division; I=staining of septal disc, Y=staining of septum split into a Y shape, X=staining of septum split into an X shape. Top row: differential interference contrast images, middle row: fluorescence images, lower row: interpretive diagrams. Images have been rotated for ease of comparison. ( c ) Percentages of organisms exhibiting incomplete or complete septa, or complete split septa ( n =219, organisms either isolated or coadhered in pairs; other: staining in an X or indistinct shape). ( d ) Cell volume in relation to splitting and septal state—newly septated cells that are yet to split have a lower volume than others. Full size image In some cases, a ring of more brightly stained material was observed to surround the partially split septum ( Fig. 2 and Supplementary Movie M1 ). Such material is attributed to the piecrust discovered by AFM imaging. Analysis of 35 single cells and 92 pairs of cells (total 219) from 9 fields acquired in 3 separate experiments in which samples were stained immediately after being returned to BHI (Ser+) showed that only about 10% had a complete septum but were yet to split ( Fig. 2c ), suggesting that the stage between septum completion and splitting is brief and that the cells spent the rest of the cycle either in making the septum or expanding and remodelling peptidoglycan in the transition from pseudo-hemisphere to sphere. Of 328 individually distinguishable sacculi or sacculi fragments in AFM images, only 3% exhibited an incomplete septum. This is likely, in part, because of masking of the incomplete septum by peripheral cell wall in many cases. Cell volumes, as expected ( Fig. 2d ), were found to be smallest for hemispherical cells that were yet to split from each other. Peptidoglycan features can specify division planes S. aureus (SH1000) sacculi exhibit one or more circular bands that would encircle the organism equatorially or at a slight offset ( Fig. 1 and Supplementary Figs S1–S4 ). Less-distinct bands, ribs, are interpreted to be the remnants of the more prominent piecrust features that would have surrounded the septum of a previous division. The piecrust feature is likely to have been split into two during septal scission. In cases in which more than one band is present, they are approximately perpendicular. AFM images of small fragments of sacculi reveal details of cross and T junctions between these features ( Fig. 3 ). Cross-junctions are formed when a piecrust bisects the rib, a piecrust remnant from a previous generation. T junctions are formed as such cross-junctions are cut when the piecrust is severed during the splitting phase of the cell cycle. 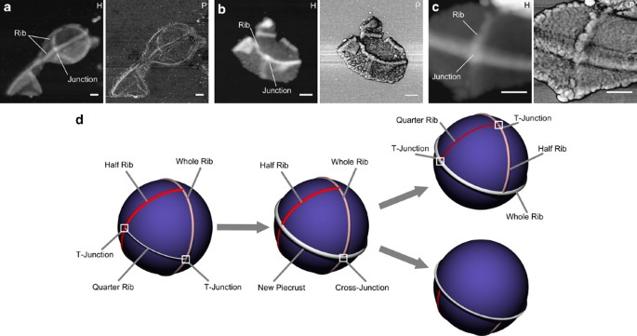Figure 3: Structural inheritance of division plane choice through peptidoglycan ribs. AFM images consist of height (H) and phase (P). (a) Broken sacculus showing ribs and a cross-junction, (b) small sacculus fragment showing details of T junction, (c) small sacculus fragment showing ribs and junction alongside ring and knobble peptidoglycan architectures, (d) Location and remodelling of piecrust and rib features through the division cycle, resulting in T and cross-junctions. A new piecrust is formed in the plane of the quarter rib; this is then split in two as the cells divide, leading to a revised rib pattern that specifies the next round of division. Colour has been used to facilitate the following of features through the process. Scales (a) bar 250 nm, H 150 nm, P 45°; (b) bar 250 nm, H 60 nm, P 20°; (c) bar 250 nm, H 100 nm, P 8°. Figure 3: Structural inheritance of division plane choice through peptidoglycan ribs. AFM images consist of height (H) and phase (P). ( a ) Broken sacculus showing ribs and a cross-junction, ( b ) small sacculus fragment showing details of T junction, ( c ) small sacculus fragment showing ribs and junction alongside ring and knobble peptidoglycan architectures, ( d ) Location and remodelling of piecrust and rib features through the division cycle, resulting in T and cross-junctions. A new piecrust is formed in the plane of the quarter rib; this is then split in two as the cells divide, leading to a revised rib pattern that specifies the next round of division. Colour has been used to facilitate the following of features through the process. Scales ( a ) bar 250 nm, H 150 nm, P 45°; ( b ) bar 250 nm, H 60 nm, P 20°; ( c ) bar 250 nm, H 100 nm, P 8°. Full size image Distribution of aging peptidoglycan in a growing population The internal sacculus rib structures also denote sectors of cell wall inherited from different generations. To investigate this phenomenon, cells were grown in BHI (Ser+), then in BHI (Ser−) for 25 min (about one division cycle), making 25 min worth of synthesized peptidoglycan accessible to the vancomycin label, a novel means of pulse labelling, before being returned to BHI (Ser+) and sampled and labelled at 15 min intervals. Images of cells sampled immediately (0 min) showed labelling of nascent material ( Fig. 4 ). After 30–60 min, the specificity of the stain for nascent material was diminished and patches of well-labelled material were visible away from the septum ( Fig. 4 ). At time points of 60 min or more, the cells labelled with qualitatively less intensity (compared with the background). This can be accounted for by the anticipated loss of terminal D -alanine residues and the incorporation of new material containing D -serine, preventing vancomycin from binding [28] . 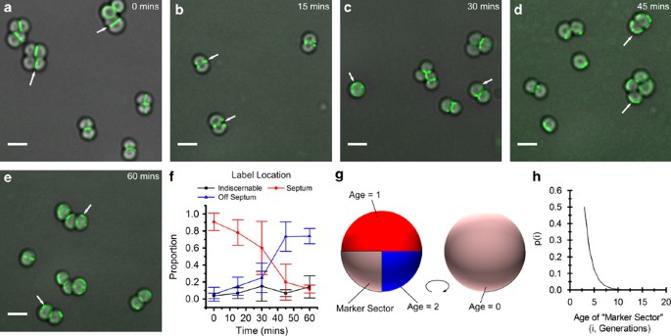Figure 4: Peptidoglycan sectoring reveals population heterogeneity. (a–e) Combined fluorescence/differential interference contrast images of vancomycin-labelledS. aureusafter growth in BHI (Ser+) following 25 min growth in BHI (Ser−). The specificity of the stain for nascent material is progressively reduced and patches of older material synthesized while the bacteria were in BHI (Ser−) are increasingly apparent away from the septum (see arrows). Scale bar: 2 μm. (f) Quantification labelling localization after incubation in BHI (Ser−). Error bars show standard deviation,n=1,584 (all time points). (g) Diagram of the 'front' and 'back' of the cell showing sectoring, illustrating that one-eighth of the cell wall is more than two generations old. (h) The probability of an organism retaining one-eighth of the cell wall from a particular previous generation: p(i). Figure 4: Peptidoglycan sectoring reveals population heterogeneity. ( a – e ) Combined fluorescence/differential interference contrast images of vancomycin-labelled S. aureus after growth in BHI (Ser+) following 25 min growth in BHI (Ser−). The specificity of the stain for nascent material is progressively reduced and patches of older material synthesized while the bacteria were in BHI (Ser−) are increasingly apparent away from the septum (see arrows). Scale bar: 2 μm. ( f ) Quantification labelling localization after incubation in BHI (Ser−). Error bars show standard deviation, n =1,584 (all time points). ( g ) Diagram of the 'front' and 'back' of the cell showing sectoring, illustrating that one-eighth of the cell wall is more than two generations old. ( h ) The probability of an organism retaining one-eighth of the cell wall from a particular previous generation: p(i). Full size image A theoretical consequence of division on sequentially orthogonal planes by S. aureus is the sectoring of peptidoglycan into segments constituting ½, ¼ or 1/8 of the cell. The redistribution of labelable material synthesized during growth in BHI (Ser−) at later time points during growth in BHI (Ser+) is a result of this, and was apparent as patches of stained material ( Fig. 4a–f ). A simple population model ( Fig. 4g,h and Supplementary Movie M2 ) was developed to show how sectors of peptidoglycan from previous generations are distributed across the current one. After three generations, all the cell walls in a population consist of ½ material from the current division (age=0), ¼ from the second most recent (age=1) and 1/8 from the division before (age=2). The remaining 1/8 is from a previous division (age>2). The probability of an organism having this one-eighth of material at age i (in integer generations) is described by the following function: where i >2, i < n −1 and n >3, with n being the number of generations for which the cells have been dividing, in practice tending to infinity. The means by which Staphylococci can coordinate division on orthogonal planes in a manner distinct from the E. coli Δ rodA mutant in which the Min system is used ( Fig. 5 ) is a long-standing question, as is the way in which peptidoglycan is architecturally arranged and remodelled through growth and division in the Staphylococcal cell wall. 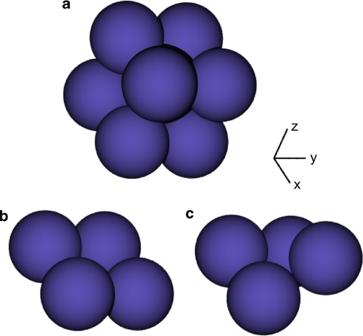Figure 5: Division in more than one plane. (a) Division in three proscribed planes leading to clusters (for example,Staphylococcus,Sarcina), the disordered clumping ofStaphylococcusis caused by coattachment, rather than division; (b) Division in two proscribed planes leading to tetrads (for example,Pediococcus); (c) Division in two planes in which the second plane is not proscribed and is free to rotate (for example,E. coliΔrodAmutant). Figure 5: Division in more than one plane. ( a ) Division in three proscribed planes leading to clusters (for example, Staphylococcus , Sarcina ), the disordered clumping of Staphylococcus is caused by coattachment, rather than division; ( b ) Division in two proscribed planes leading to tetrads (for example, Pediococcus ); ( c ) Division in two planes in which the second plane is not proscribed and is free to rotate (for example, E. coli Δ rodA mutant). Full size image AFM imaging revealed large piecrust structures that are retained as ribs as the cell undergoes cycles of division. Also observed were ring and knobble surface architectures. The similarity between the diameter of the piecrust as measured by AFM and the diameter of whole cells as measured by differential interference contrast microscopy shows that these features are not the leading edge of the septum, a marked difference from B. subtilis , the septum of which has somewhat raised leading and lagging edges [18] . Such features may also be associated with 'bridge' regions of cell wall previously observed by cryo-transmission electron microscopy of pure S. aureus peptidoglycan [29] . The use of a pure peptidoglycan sample, as opposed to a whole cell, demonstrates that ring structures are made of peptidoglycan, not protein or teichoic acid. As it is known from previous work that nascent cell wall adopts the ring structure [3] , [26] , the knobbles must be formed by remodelling of rings. The knobble structure has not previously been observed in whole cells by AFM or electron microscopy in which 'network' or 'honeycomb' structures, possibly combinations of peptidoglycan, protein and teichoic acids, have been reported, in addition to concentric rings [3] , [21] , [23] , [26] . The presence of rarely observed hybrid ring-knobble architectures suggests that remodelling occurs by lateral expansion of peptidoglycan, by discontinuous autolysis along the rings. In no case was a high, crystalline degree of order observed. This, coupled with the heterogeneity of the material, explains why deriving X-ray structures of peptidoglycan has presented such a challenge for researchers [30] . The architecture of S. aureus is very different from that of B. subtilis [18] , illustrating that peptidoglycan is able to assume different architectural forms to permit the full range of bacterial shapes and growth modes. Fluorescent vancomycin labelling showed that, when dividing, cells form a ring of peptidoglycan, followed by a septal disc creating hemispherical daughter cells that then split into an X or Y conformation before the cells expand further to a more spherical shape. During this splitting and stretching, the rings observed by AFM are most likely to be remodelled into knobbles. The Y conformation is characteristic of eccentric attachment of daughter cells, as previously observed by phase contrast [1] and electron microscopy [19] , and allows the organisms to form irregular bunched clusters [1] rather than the more regular arrangements adopted by other genera that divide on orthogonal planes ( Fig. 5 ): cuboidal packets (for example, Sarcina ) or rectilinear grid arrangements (for example, Pediococcus ) [3] . Effective pulse labelling of peptidoglycan using serine substitution in the crosslinking peptide allowed the inheritance of cell wall to be tracked in aging cells. The inherited peptidoglycan has covalently attached proteins of a blend of types suited to the environment that the organism was in at the time of incorporation [31] . Dynamic environmental conditions, such as those encountered during pathogenesis, will lead to alterations in surface protein expression. Thus, cells may also inherit a surface protein complement with heterogeneity within the population, especially of those proteins only attached during septum formation [32] , [33] . Such population-wide heterogeneity may provide a selective advantage in the ever-changing complex interaction between pathogen and host. Dependent on the mode of peptidoglycan, and associated linked protein, incorporation during growth and division, such population heterogeneity may be more widespread among the bacteria. For instance, Bacilli are known to retain pole material over several generations [34] . For cells that were not pulse labelled, the measured increase in volume from hemispherical to spherical cells demonstrates that, as suggested [35] , volume increases, ultimately doubling, after the scission of the septum, leading to an increase in surface area. This occurs without further synthesis of peptidoglycan [27] . The cells must therefore remodel the septal peptidoglycan under the constraint that the hemispherical cell must double in volume [36] , requiring an alteration in peptidoglycan density. If, hypothetically, the cell wall were not present, then the hemispherical daughter cells would become spheres of half the parent volume so as to minimize surface energy. In practice, the cell experiences pressurization because of continuous synthesis and acquisition of osmolytes, which is presumably uninterrupted by division and which drives the volume increase. The radius of the cell at what was the septum may be braced by the piecrust bands of peptidoglycan observed by AFM, preventing collapse to a smaller sphere and mandating expansion of the nascent, septal wall. It is known from scanning electron microscopy imaging of sister cells that the ring architecture is associated with a new cell wall [3] . The transition from rings to knobbles must therefore be a result of irreversible, inelastic changes in peptidoglycan morphology as a result of autolysis of covalent bonds (as isolated sacculi do not revert to pseudo-hemispherical conformation). It has already been shown that N -acetylglucosaminidase activity is responsible for processing of glycan strands in S. aureus and it may be this activity that allows the growth without synthesis, through hydrolysis of nascent septal peptidoglycan [16] . The location of the next division plane must be orthogonal to the previous two, both of which are denoted by retained ribs originating from previous divisions, a whole rib from the most recent and a half rib from the second most recent. The third most recent division plane, also the plane of the next active division, is demarked by a quarter rib that is uniquely bounded by two T junctions. The ribs therefore encode enough information to determine the location of the next plane of division and so maintain the characteristic three-plane sequence ( Fig. 3 ). To execute division, the cell must recruit the proteins of the divisome to the nascent septal ring. Spatial regulation of proteins in bacteria is not well understood and is thought to generally occur by 'diffusion and capture' [37] . This begets the question of how the captor protein was localized: what are the 'ultimate cues' that initiate the binding together of the divisome? The candidates for this are oscillators (such as those established by the Min system in E. coli [4] , [38] and Neisseria [39] ), membrane curvature (recognized by B. subtilis DivIVA [40] ) and epigenetic inheritance of already localized proteins (such as TipN in Caulobacter crescentus [41] , [42] , although this protein is not part of the divisome). No such systems are known to exist in S. aureus . There is no Min system or homologue, and proteins capable of recognizing membrane curvature have not been characterized, other than FtsZ, which has a complex membrane interaction in that it can both recognize and modify curvature [43] , [44] . The nucleoid occlusion (Noc) protein prevents division through a nucleoid in B. subtilis [45] by presumed direct or indirect interaction with FtsZ, and the kinetics of division as a result of the timing of replication of Noc-binding sites on the chromosome [46] , but does not position the nucleoid so as to set septum location, and as such is not an 'ultimate cue'. A Noc homologue is present in S. aureus but is of currently unknown function [47] . We have no means of specifically removing ribs without disrupting peptidoglycan integrity, which makes absolute determination of the mechanism by which ribs can be recognized by the divisome problematical. The organism must determine the location of the active division plane by exclusion of the two most recent planes, or by recognition and alignment with the quarter rib from the third most recent plane. Ribs may either be recognized by a ligand–receptor-type interaction between the mostly uncharacterized divisome and the distinct peptidoglycan architecture in the ribs, in the rib junctions, or by recognition of the distinct curvature that is imprinted on the cytoplasmic membrane by ribs and inter-rib junctions. The plane containing the quarter rib has the longest circumference, as there is the minimum protrusion of peptidoglycan impinging on the cytoplasmic membrane (by direct physical contact or by the periplasm [29] ), and thus the largest average radius of curvature. This may single it out for recognition. The architectural features and means of remodelling peptidoglycan during division have evolved to solve the requirements of division in three planes and may be common to other bacterial geometries in which division plane selection is proscribed [3] . The piecrust/rib and sectoring systems initiate a new class of structural inheritance and may indicate that epigenetic information is more important in organisms that reproduce by binary fission than previously thought, given that inherited structures constitute such a large proportion of total material in the mature cell. Strains and growth conditions S. aureus (SH1000) were grown in BHI (Oxoid CM0225) at 37 °C with agitation at 250 r.p.m. Preparation of S. aureus sacculi Organisms were collected at exponential (OD 600 ∼ 0.4) or stationary phase ( ∼ 12 h growth), boiled for 7 min, broken by FastPrep and subsequently purified as previously described [11] . Broken cells were suspended in 5% (w/v) SDS at 55 °C in a 15 ml Falcon tube and boiled in a water bath (100 °C) for 25 min. Insoluble material was collected by centrifugation at room temperature ( ∼ 23 °C). This process was repeated using 4% SDS and a 15 min boil. The resulting pellets were washed six times with distilled water (60 °C). They were then resuspended in Tris-HCL (50 mM, pH 7) with 2 mg ml −1 Pronase and incubated at 60 °C for 90 min. This was followed by a single distilled water wash as before. Pellets were resuspended in 250 μl hydrofluoric acid and incubated overnight at 4 °C, before being washed five times in distilled water at room temperature and then resuspended in Tris-HCL (50 mM, pH 7) for storage at −20 °C. AFM of S. aureus sacculi Before imaging, sacculi samples were tip sonicated three times for 30 s to break up flocculates, adjusted to an appropriate working dilution with Milli-Q water and then dried onto freshly cleaved mica with a stream of nitrogen before being washed three times with Milli-Q water, then dried again as before. AFM was carried out in 'Tapping Mode' using silicon tips (Olympus) in ambient conditions using a Multimode or Dimension AFM with an Extended Nanoscope IIIa controller (Veeco Instruments). Images were line corrected using the 'Level rows using intersections of given lines' function, flattened by plane subtraction and scales set for optimal contrast in Gwyddion (version 2.8 or greater). Scale bars were added using ImageJ (1.41o). The outer diameter of a rib/piecrust was determined by measuring the length of the long and short axes of the region enclosed by it, which specified an ellipse, then calculating the diameter of a circle of equivalent area. Labelling of nascent peptidoglycan with vancomycin A culture of SH1000 was grown overnight in BHI containing 125 mM d-serine (Sigma S4250), diluted into the same medium to an OD 600 of ∼ 0.01, then grown to an OD 600 of ∼ 0.4, corresponding to the mid-exponential phase. The culture was then transferred by centrifugation and resuspension into BHI (without D -serine) and grown for 25 min, finally transferred into BHI containing 125 mM D -serine once more for further growth. Samples were extracted at 15 min intervals and labelled with a 1:1 mix of vancomycin (Sigma V-2002):vancomycin-BODIPY (Invitrogen V-34850) at 0.5 or 1 μg ml −1 , before being cooled to 4 °C and washed twice with distilled water. Fluorescence microscopy Cells were fixed (0.42 ml 15% v/v formaldehyde, 2.08 ml PBS, 0.5 μl 25% v/v glutaraldehyde), mounted on poly- L -lysine-coated slides and then imaged using a Deltavision deconvolution microscope (Applied Precision), deconvolved and adjusted for optimal contrast using Softworx (3.5.1). Cell counting was conducted using ImageJ (1.41o); organisms in large clumps were not counted, as the distribution of the stain could not be determined. Scale bars were added using ImageJ (1.41o). Cell volume calculations Measurements were obtained using Softworx (3.5.1) and were limited to single organisms or pairs of organisms separate from large clumps. In cases in which daughter cells had not split, volume was calculated assuming a hemispherical shape from measured dimensions ( Fig. 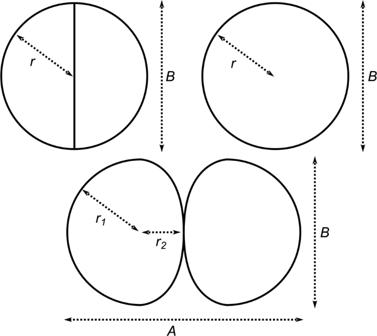Figure 6: Dimensions measured for volume calculations and radii of pseudo-hemispherical cells. See equations (2,3,4,5). 6 ): Figure 6: Dimensions measured for volume calculations and radii of pseudo-hemispherical cells. See equations (2,3,4,5). Full size image For completely separated cells with no visible septum, volume was calculated assuming a spherical shape: In cases in which daughter cells had partially split (X or Y), volume was calculated assuming a pseudo-hemispherical shape, in cases in which half of the cell is hemispherical and the other half is ellipsoid: All pairs of cells have identical volumes on the basis of these measurements, but each cell may be separately classified depending on whether it had an incomplete septum. How to cite this article: Turner, R. D. et al . Peptidoglycan architecture can specify division planes in Staphylococcus aureus . Nat. Commun. 1:26 doi: 10.1038/ncomms1025 (2010).